Molecular mechanics of mineralized collagen fibrils in bone Bone is a natural composite of collagen protein and the mineral hydroxyapatite. The structure of bone is known to be important to its load-bearing characteristics, but relatively little is known about this structure or the mechanism that govern deformation at the molecular scale. Here we perform full-atomistic calculations of the three-dimensional molecular structure of a mineralized collagen protein matrix to try to better understand its mechanical characteristics under tensile loading at various mineral densities. We find that as the mineral density increases, the tensile modulus of the network increases monotonically and well beyond that of pure collagen fibrils. Our results suggest that the mineral crystals within this network bears up to four times the stress of the collagen fibrils, whereas the collagen is predominantly responsible for the material’s deformation response. These findings reveal the mechanism by which bone is able to achieve superior energy dissipation and fracture resistance characteristics beyond its individual constituents. Bone is a remarkable hierarchical biomaterial ( Fig. 1a ) that has two major constituents, soft collagen protein and much stiffer apatite mineral [1] , [2] . During the formation of bone, collagen molecules assemble into fibrils, which are mineralized via the formation of apatite crystals. Although larger-scale bone structures differentiate depending on bone type and species, the structure of mineralized fibrils is highly conserved across species and different types of bone, and hence act as the bone’s universal elementary building block [3] , [4] , [5] , [6] . The hierarchical structure of bone enables it to be a light-weight material that can carry large loads, and combines the toughness of inorganic material and the flexibility of protein-based tissues [7] , [8] , [9] , [10] , [11] , [12] . Previous studies based on mechanical models have uncovered key mechanistic features of bone as well, eluded to the role of mineral platelets in strengthening the material [13] , [14] , [15] , [16] , [17] , [18] . At the nanoscale, the interactions between collagen molecules and the mineral hydroxyapatite (HAP), and as well as the amount of mineral, are known to have a significant role in providing strength and toughness to the bone (or lack thereof, in disease states). In this paper we focus on the structure and mechanics of mineralized collagen fibrils, as it is universally found in many types of bone. Collagen–HAP composites are not only the basic building blocks of the human bone, but they are also amongst the most abundant class of biomineralized materials in the animal kingdom (found in the skeletal system, teeth or antler) [1] , [2] . 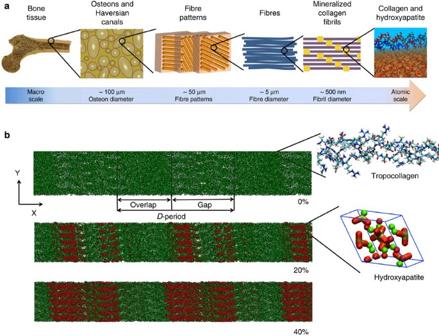Figure 1: Bone structure and model development. (a) Hierarchical structure of bone ranging from the macroscale skeleton to nanoscale collagen (green) and HAP (red). (b) Collagen microfibril model with 0% mineralization (inset shows the collagen triple-helix structure), 20% mineral content (inset shows a HAP unit cell) and 40% mineral content. The HAP crystals are arranged such that the c axis of crystal aligns with the fibril axis. Ca atoms plotted in green, OH groups plotted in red and white, and the tetrahedron structure visualizes the PO4group. The left three images in panelataken from Launeyet al.65 Figure 1: Bone structure and model development. ( a ) Hierarchical structure of bone ranging from the macroscale skeleton to nanoscale collagen (green) and HAP (red). ( b ) Collagen microfibril model with 0% mineralization (inset shows the collagen triple-helix structure), 20% mineral content (inset shows a HAP unit cell) and 40% mineral content. The HAP crystals are arranged such that the c axis of crystal aligns with the fibril axis. Ca atoms plotted in green, OH groups plotted in red and white, and the tetrahedron structure visualizes the PO 4 group. The left three images in panel a taken from Launey et al . [65] Full size image Although the structure of bone and its mechanical properties have been well-studied, the knowledge about how collagen fibrils and HAP crystals interact at the molecular scale, and how they deform as an integrated system under external stress are not well understood. Developing a deeper understanding of the properties of bone from the level of its building blocks requires a thorough investigation of the interplay of the organic protein molecules with the mineral crystals. This, in turn, requires an atomistic-level investigation of the properties of the organic–inorganic interfaces [19] , [20] and its correlation with the overall mechanical behaviour. Several attempts have been made to develop a molecular model of bone, but those studies fell short to providing a full three-dimensional, chemically and structurally accurate model of the interactions of collagen with the mineral phase [21] , [22] , [23] , [24] . Coarse-grain models [25] of nascent bone showed that the mineral crystals provide additional strength and also increases the Young’s modulus and fracture strength. Although these models provided some insight into the mechanics of bone, they failed to capture atomic-scale mechanisms, did not reach higher mineralization levels, and did not allow for a direct comparison with experimental work (for example, in situ x-ray analysis of bone deformation [1] , [2] , [3] , [4] , [5] , [6] ). The coarse-grain description of nascent bone [25] is a highly simplified two-dimensional model and relies on empirically derived mechanical parameters, which were not directly derived from fundamental principles of chemical interactions. The model also neglected the details of the shape or distribution of the mineral platelets, which is likely to have an important impact on the mechanical properties of the material. In this paper we develop a three-dimensional, full-atomistic mineralized collagen microfibril model and perform tensile tests at various stress levels, to identify key deformation mechanisms. We find that as the mineral density increases, the tensile modulus increases successively, and is significantly larger than that of pure collagen fibrils. By comparing stress and strain fields associated with different mineral content and applied stress, we find that the mineral crystals carry about four times the stress compared with collagen, whereas the protein phase carries the bulk of deformation. These findings reveal the mechanism by which bone carries load at the nanoscale, where the district distribution of stress and strain between collagen and HAP enables a mechanism of great energy dissipation and resistance to fracture that overcomes the intrinsic limitations of the constituents and amplifies their superior properties. Mineralized microfibril model We apply an in silico mineralization scheme based on a Monte Carlo approach, and identify molecular structures of nascent bone for different mineral densities, from 0% (pure collagen microfibril, see Fig. 1b for model details) to 40% (highly mineralized collagen fibril). As shown in Fig. 2a , the mineral is deposited predominantly in the gap region along the fibril axis, with sparse deposition in the overlap region. 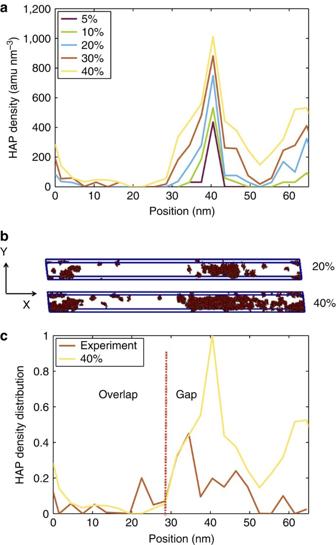Figure 2: Mineral distribution in the collagen microfibril at different mineralization stages. (a) Distribution of HAP along the collagen fibril axis. The data shows that the maximum amount of HAP is found in the gap region (between 30 and 50 nm). (b) Spatial distribution of HAP in the unit cell for 20 and 40% mineral density. (c) HAP density distribution along the fibril axis for the 40% case normalized (same data as depicted in panela) compared with experimental data26. The comparison confirms that maximum deposition is found in the gap region. Figure 2b shows a detailed analysis of the distribution of mineral crystals for 20 and 40% mineral densities. We perform a direct comparison with experimental results that reported the distribution of mineral density as a function of the fibril axis [26] , and plot the mineral distribution of 40% case normalized to its maximum value along with experimental results along the fibril axis ( Fig. 2c ). In good agreement with a rich set of experimental data [1] , [2] , [3] , [4] , [5] , [6] , [26] , [27] in the mineralized microfibril models with varying densities (5, 10, 20, 40%, and so on), the mineral deposition occurs primarily in the gap region. This observation is also consistent with the experimental finding [26] that the mineral nucleation point is close to the carboxy terminus (in the first section of the gap region, immediately after the gap/overlap transition). As discussed by Nudelman et al . [26] , the main reason is the high concentration of positive charge, which attract negatively charged peptides, in turn responsible for onset of mineralization. Our in silico mineralization process is not driven by electrostatic interactions (see Methods ), but rather relies on a geometric argument, driven by the void space available within the virgin (non-mineralized) collagen fibril. This may suggest that in the in vivo mineralization process there could be concurrent mechanisms that lead to the nucleation in the C-terminal region. Along with the concentration of positive net charges, the C terminus region also features larger void spaces in the collagen packing, which makes this region the preferred site for mineral nucleation. We find that the 40% mineral-density case shows more mineral deposition in the gap region compared with experimental data [26] . This could be due to the fact that in the experimental work, the mineral density profile is measured for collagen that is mineralized for 24 h. Our model shows that the size of the mineral platelets in the gap region is ~15 × 3 × 1.6 nm 3 (for the case of 40% mineral density). This is in good agreement with experimental work that has shown that the size of mineral platelets is 15–55 × 5–25 × 2–3 nm 3 ( [26] , [27] , [28] ). We note that the models are based on a periodic unit cell of a collagen microfibril with approximate dimensions of 67.8 × 4 × 2.7 nm (see further discussion regarding structural aspects below). It is possible that the mineral phase can span several unit cells and, hence, forms larger size HAP platelets in vivo , explaining the larger range of values. Figure 2: Mineral distribution in the collagen microfibril at different mineralization stages. ( a ) Distribution of HAP along the collagen fibril axis. The data shows that the maximum amount of HAP is found in the gap region (between 30 and 50 nm). ( b ) Spatial distribution of HAP in the unit cell for 20 and 40% mineral density. ( c ) HAP density distribution along the fibril axis for the 40% case normalized (same data as depicted in panel a ) compared with experimental data [26] . The comparison confirms that maximum deposition is found in the gap region. Full size image Mechanical testing We carry out tensile tests on non-mineralized (0%), 20 and 40% mineral density samples ( Fig. 3a ). As observed from Fig. 3b , as the mineral content increases, the stress–strain behaviour of the mineralized collagen microfibril also changes compared with pure collagen fibrils, with the mineralized cases showing an increasingly higher modulus as higher mineral densities are reached. To quantify the variation of the modulus for different strain levels, we plot the modulus as a function of strain as shown in Fig. 3c . The 0% case has an initial modulus of 0.5 GPa at a load less than 20 MPa, and increases to 1.1 GPa as the stress increases to 100 MPa. For larger deformation, the modulus approaches 2 GPa. These moduli are well within the range of values reported for collagen fibrils under tensile loading using both experiment and simulation [29] , [30] . For the 20% mineral-density case, the initial modulus is 1.3 GPa (stress less than 20 MPa) and increases to 2.7 GPa at 100 MPa. This shows that even a relatively small mineral content severely alters the stress–strain behaviour of collagen microfibril model and increases its modulus by ~150%. Similarly, the 40% mineral-density case has an initial modulus of 1.5 GPa, approaching 2.8 GPa. For stresses at 100 MPa, the 20 and 40% mineral-density cases have very similar tangent moduli. However, as shown in Fig. 3c , as the strain increases beyond 10%, the modulus for the 40% mineral-density case also increases, indicating that at higher strains the mineral content provides additional stiffness to the collagen–HAP composite. The moduli identified here for the cases with 20 and 40% mineral content is consistent with a recent experimental study [31] , which showed that mineralized collagen fibrils from antler had a modulus of 2.38±0.37 GPa for strain less than 4%. 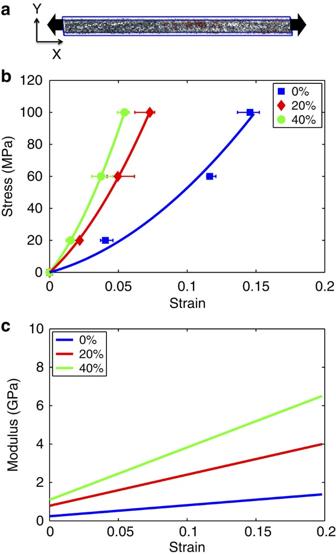Figure 3: Mechanical properties of collagen fibrils at different mineralization stages. (a) Fibril unit cell with mineral content used to perform tensile test by measuring stress versus strain. (b) Stress–strain plots for non-mineralized collagen fibril (0%), 20% mineral density and 40% mineral-density cases. (c) Modulus versus strain for 0, 20 and 40% mineral density showing an increase in modulus as the mineral content increases. The error bars inbare computed from the maximum and minimum values of the periodic box length along the x direction at equilibrium. Figure 3: Mechanical properties of collagen fibrils at different mineralization stages. ( a ) Fibril unit cell with mineral content used to perform tensile test by measuring stress versus strain. ( b ) Stress–strain plots for non-mineralized collagen fibril (0%), 20% mineral density and 40% mineral-density cases. ( c ) Modulus versus strain for 0, 20 and 40% mineral density showing an increase in modulus as the mineral content increases. The error bars in b are computed from the maximum and minimum values of the periodic box length along the x direction at equilibrium. Full size image Nanoscale deformation mechanisms To understand the deformation mechanism for mineralized and non-mineralized samples at different deformation states, we compute the deformation fields within the fibrils. We observe that as the loading increases, there is no significant movement or coalescence of the HAP crystals in the gap region when the loading increases from 20–100 MPa. However, for the 0% case, the collagen molecule undergoes significant deformation in the gap region as the applied stress increases. We compute the deformation in the collagen microfibril for all three cases at applied stresses of 20, 60 and 100 MPa. As seen in Fig. 4 , the gap-to-overlap ratio for 0% case increases with the applied stress, indicating that for pure collagen the gap region deforms significantly compared with the overlap region to accommodate the external load. This behaviour is consistent with earlier tensile tests on collagen microfibril [30] . Clearly, the presence of HAP alters the deformation mechanism of the collagen fibril. For the 20% mineral-density case, the gap-to-overlap ratio is nearly constant for increases in applied stress, whereas for the 40% case the gap-to-overlap ratio decreases as the applied stress increases. This shows that a higher mineral content leads to more deformation in the overlap region compared with the gap region, where the interaction between HAP and collagen limits the deformation within collagen molecules. It has been previously suggested that the interaction between mineral and collagen is mainly due to electrostatic interactions and hydrogen bonding [32] . An analysis of the number of hydrogen bonds between the mineral and collagen in the gap region shows that the mineralized case has ~18–20% more hydrogen bonds compared with the non-mineralized case, where the hydrogen bonding occurs solely between the chains within the collagen molecule. Another important mechanism of load transfer between collagen and HAP is due to salt bridges (electrostatic interactions between charged moieties). Although in the non-mineralized fibril this type of non-covalent interaction is minor, it becomes rather important in the mineralized samples. As shown in Fig. 5 , the vast majority of salt bridges are formed within the mineral crystals; however, a non-negligible number of salt bridges are formed between mineral crystals and collagen, providing an effective load transfer mechanism between the mineral and organic phase that also enhances energy dissipation. This further explains our finding that the overlap region deforms more compared with gap region in the mineralized cases, a clear distinction from the mechanics of pure collagen fibrils. 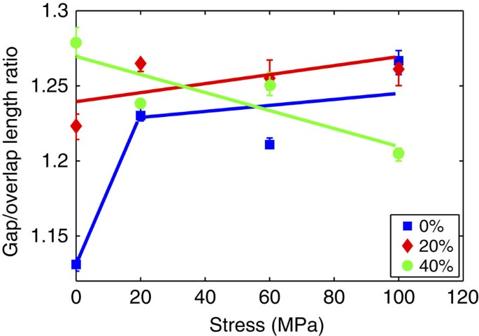Figure 4: Variation of the gap-to-overlap length ratio as the applied stress increases for different HAP contents. The deformation mechanism of non-mineralized collagen fibrils is molecular straightening in the crimped and loosely packed gap region (at small deformations), followed by molecular stretching (across the fullD-period) at larger deformations. These mechanisms result in an initial increase in the gap/overlap ratio, which then remains constant, as is observed in the non-mineralized model reported here (where the gap/overlap ratio increases from 0–20 MPa stress). In contrast, in the mineralized cases the deformation mechanism is radically changed. Indeed, in the lower mineralized model (20% HAP) we do not observe any significant change in the gap/overlap ratio, suggesting that theD-period deforms rather uniformly, due to the stiffening effect of HAP mainly in the gap region. However, in the highly mineralized model (40% HAP), the trend is inverted, where the gap/overlap region decreases, suggesting that in this case the gap region is stiffer and that deformation takes place primarily in the overlap region. The error bars are obtained from the maximum and minimum values of the periodic box length along the x direction obtained after equilibration of each sample, which is utilized to compute the gap and overlap lengths. Figure 4: Variation of the gap-to-overlap length ratio as the applied stress increases for different HAP contents. The deformation mechanism of non-mineralized collagen fibrils is molecular straightening in the crimped and loosely packed gap region (at small deformations), followed by molecular stretching (across the full D -period) at larger deformations. These mechanisms result in an initial increase in the gap/overlap ratio, which then remains constant, as is observed in the non-mineralized model reported here (where the gap/overlap ratio increases from 0–20 MPa stress). In contrast, in the mineralized cases the deformation mechanism is radically changed. Indeed, in the lower mineralized model (20% HAP) we do not observe any significant change in the gap/overlap ratio, suggesting that the D -period deforms rather uniformly, due to the stiffening effect of HAP mainly in the gap region. However, in the highly mineralized model (40% HAP), the trend is inverted, where the gap/overlap region decreases, suggesting that in this case the gap region is stiffer and that deformation takes place primarily in the overlap region. The error bars are obtained from the maximum and minimum values of the periodic box length along the x direction obtained after equilibration of each sample, which is utilized to compute the gap and overlap lengths. 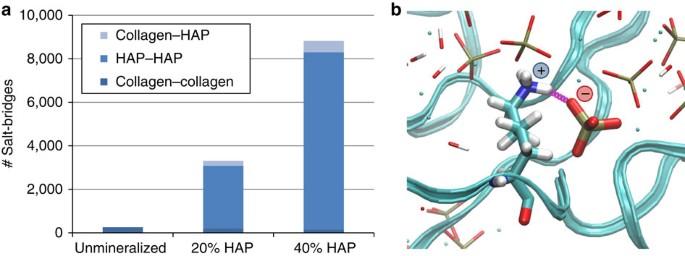Figure 5: Salt bridges in mineralized and non-mineralized collagen fibrils. (a) Number of salt bridges per unit cell. In the non-mineralized model, the number of salt bridges is ~260, due to interactions between charged side chains of collagen: lysine (+), arginine (+), glutamic acid (−) and aspartic acid (−). In the mineralized models, there is a high number of mineral–mineral salt bridges, due to the fact that the moieties forming HAP are highly charged: Ca2+, PO43−and OH−. Salt bridges are also found relevant between collagen and mineral phase (about 220 and 520 in 20% HAP and 40% HAP case, respectively), contributing to the increase in mechanical properties of mineralized fibrils. Panelbshows an example of salt bridge between a lysine (+) side chain and mineral PO43−group. Full size image Figure 5: Salt bridges in mineralized and non-mineralized collagen fibrils. ( a ) Number of salt bridges per unit cell. In the non-mineralized model, the number of salt bridges is ~260, due to interactions between charged side chains of collagen: lysine (+), arginine (+), glutamic acid (−) and aspartic acid (−). In the mineralized models, there is a high number of mineral–mineral salt bridges, due to the fact that the moieties forming HAP are highly charged: Ca 2+ , PO 4 3− and OH − . Salt bridges are also found relevant between collagen and mineral phase (about 220 and 520 in 20% HAP and 40% HAP case, respectively), contributing to the increase in mechanical properties of mineralized fibrils. Panel b shows an example of salt bridge between a lysine (+) side chain and mineral PO 4 3− group. Full size image Stress and strain distribution in non-mineralized and mineralized fibrils To understand the distribution of stress inside the microfibril, we compute the stress distribution in the cross sectional y–z plane ( Fig. 6a ). The virial stresses [33] are computed for an applied stress of 100 MPa for 0%, 20% and 40% mineral-density cases, respectively. To visualize and quantify the stresses in the unit cell, we compute the principal stresses for a region with a finite thickness of 15 Å in the x direction. For the 0% case we choose the overlap region, and for the 20 and 40% mineral-density cases we chose the gap region for principal stress computation. As observed from Fig. 6a , the 0% case has a nearly uniform stress distribution with maximum stresses reaching ~15 MPa, indicating that the collagen backbone gets stretched and the three chains take the load. The mineralized cases show higher stress in HAP compared with collagen, with maximum stress reaching 50 MPa, hence suggesting that the load is predominantly carried by the mineral phase. To validate this finding, we plot the average stress in collagen and the mineral phase for 20 and 40% mineral densities. 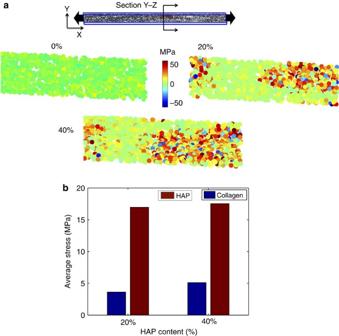Figure 6: Analysis of stress fields for different mineral contents. (a) View of the cross-section of the y–z plane of the unit cell used to perform the stress analysis. The principal stress contours for an applied stress of 100 MPa in collagen microfibril show a nearly uniform stress distribution, whereas the data for 20 and 40% mineral-density cases clearly reveals significantly higher stress regions in the HAP mineral. (b) Quantification of the overall average stress in the collagen and mineral phases at 100 MPa applied stress, showing that the mineral phase features about four times the stress level compared with collagen. Figure 6b shows that the HAP phase takes approximately four times the stress compared with collagen. This leads to the conclusion that as the mineral content increases, there is a stronger interaction between the mineral and the collagen, and that the applied load is distributed among collagen and mineral phases in a particular pattern. Figure 6: Analysis of stress fields for different mineral contents. ( a ) View of the cross-section of the y–z plane of the unit cell used to perform the stress analysis. The principal stress contours for an applied stress of 100 MPa in collagen microfibril show a nearly uniform stress distribution, whereas the data for 20 and 40% mineral-density cases clearly reveals significantly higher stress regions in the HAP mineral. ( b ) Quantification of the overall average stress in the collagen and mineral phases at 100 MPa applied stress, showing that the mineral phase features about four times the stress level compared with collagen. Full size image To quantify the strain distribution in the collagen and HAP phase, we compute the end-to-end distance for collagen molecule at 0 and 100 MPa. From the computed difference in end-to-end length for 0 and 100 MPa applied stresses, we find that the collagen phase with mineral density of 20% takes 7.3% strain, whereas for 40% mineral density the strain is 6.3%. For the HAP phase, we estimate the strain from the bulk modulus of HAP (100 GPa computed from our model, and is in good agreement with previous studies [34] ) along the x axis at an applied stress of 100 MPa. The value of strain in the HAP phase is 0.06%, which is two orders of magnitude lower than the strain in the collagen phase. These findings and our observation that the strain in collagen is lower than the total strain is in very good agreement with earlier studies [4] , [35] , and suggests that in the mineralized collagen microfibril the collagen deforms significantly more than the HAP crystals. We also compute the stress in mineral platelets from the strain values of mineral as reported in Gupta et al . [4] and using a modulus of 100 GPa. The stress in the mineral at 100 MPa applied stress is ~110 MPa. We note that the stress in the mineral is higher (by approximately two times) than the value we obtained from our model. This could be because of the fact that our model does not include extrafibrillar mineral content, and that the extrafibrillar mineral content could have an important role in stress transfer between fibrils by shear deformation as suggested earlier [4] . Mineral crystals carry more stress, whereas the collagen protein carries more deformation. This distribution of stress and strain between collagen and HAP at the nanoscale enables a mechanism of energy dissipation and, as such, resistance to fracture in bone. As observed in a recent atomistic study [23] that focused on the interface between collagen and HAP, a collagen molecule at high stress levels gets stretched and starts to uncoil, and eventually slides on the HAP surface. Our mineralized microfibril model, the deformation process at low stress levels, indicates the onset of such a deformation mechanism, where the overlap region deforms more compared with the gap region. Although available models of mineralized fibrils reflect a range of theoretical and analytical models (even if very complex), our model for the first time accounts for the full biochemistry of mineralized fibrils, as it is an all-atom molecular model. The model can easily be adapted to other collagen sequences, geometries or bone types, and is hence anticipated to have broad impact for future modelling and experimental work. As a consequence of the fundamental approach, our model is not only able to correctly predict the gross mechanical properties of mineralized fibrils, but it also allows obtaining fundamental insights on the nanoscale deformation mechanisms and on the load transfer between collagen and mineral. For example, the parameters derived from our model can be incorporated into existing analytical models [13] , [36] , [37] and can provide parameter estimates from a fundamental perspective. We specifically compare two analytical approaches reported in ( [36] , [37] , [38] ) with the simulation and experimental results [31] (details of the analytical models see Methods ). As observed from Fig. 7 , Gao’s model [37] predicts a slightly lower modulus for low mineral volume fraction and increases as the mineral volume fraction increases, but is consistent with atomistic and experimental values for high mineral volume fraction. The Halpin–Tsai bone model [36] , [38] predicts a much higher modulus compared with Gao’s model, simulation results and experimental data, as the mineral volume fraction increases. The difference between the analytical models is likely due to the fact that Gao’s model was developed from the experimental observation of the bone nanostructure, which explains the overall good agreement. Moreover, in Gao’s model the effective stiffness depends on the shear modulus G p of the collagen, which is several orders of magnitude lower than the modulus of the mineral. Hence, at low mineral volume fractions the effective modulus is likely dominated by the shear modulus and the aspect ratio of the mineral ( G p ρ 2 ). The difference between analytical models and simulations could be due to the assumption in the analytical model that minerals are rectangular blocks, and that the mineral size and shape doesn’t change in the gap and overlap regions. Therefore, one possible insight derived from this comparison is that the variation of mineral size and shape in the gap and overlap region controls the effective modulus and deformation mechanisms at the nanoscale, and must be taken into consideration. 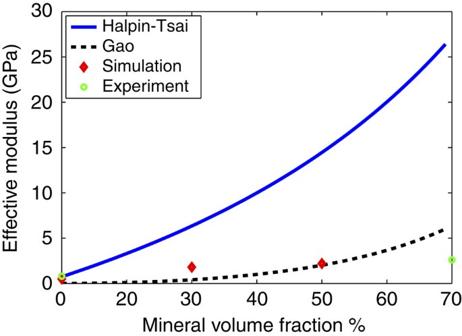Figure 7: Variation of effective modulus with respect to mineral volume fraction comparing simulation, experiment and analytical models. Comparison of analytical models by Halpin–Tsai36,38and Gaoet al.37with our simulation data and experimental results31. The analytical model by Halpin–Tsai (equations (1) and (2)) predicts a higher modulus as the mineral volume fraction increases compared with Gao’s model, simulation and experimental modulus. The Gao model (equation (3)) agrees better overall, but predicts a lower modulus for very low mineral content and deviates from the atomistic and experimental predictions for higher mineral content. Figure 7: Variation of effective modulus with respect to mineral volume fraction comparing simulation, experiment and analytical models. Comparison of analytical models by Halpin–Tsai [36] , [38] and Gao et al . [37] with our simulation data and experimental results [31] . The analytical model by Halpin–Tsai (equations (1) and (2)) predicts a higher modulus as the mineral volume fraction increases compared with Gao’s model, simulation and experimental modulus. The Gao model (equation (3)) agrees better overall, but predicts a lower modulus for very low mineral content and deviates from the atomistic and experimental predictions for higher mineral content. Full size image Our model predicts the characteristic elongated shape of mineral platelets with an ultra-small thickness on the order of a few nanometers (approximate crystal dimensions ~15 × 3 × 1.6 nm 3 ). The geometric confinement to very thin nanometer crystals has been suggested to have a critical role in achieving flaw tolerance [37] , a phenomenon that has been confirmed in full-atomistic simulation [39] . Mineral crystals at that size are no longer brittle (as they are at the macro scale, for example, classroom chalk), but instead show a highly ductile behaviour [39] . As the mineral content increases from 20–40%, the modulus increases continuously, confirming that mineral deposition leads to significant stiffening during bone formation. The detailed understanding of the mechanics of this process could be important in identifying the cellular response to changes in the mechanical microenvironment [26] , [40] , [41] , as well as for models of bone remodelling and tissue engineering [1] , [2] , [9] , [42] , [43] . The load transfer mechanism between the organic phase (collagen) and the inorganic phase (HAP) is due to electrostatic interactions, namely hydrogen bonds and salt bridges. These interactions can explain the enhanced capacity to dissipate energy as it enables a stick–slip deformation process activated at large deformation. Altogether, the mineral crystals carry more stress, whereas the collagen protein carries more deformation. This distribution of stress and strain is critical, as it takes advantage of the great stiffness of minerals and the energy dissipating capacity of collagen molecules through uncoiling of their triple helical structure, similar to sacrificial mechanisms observed at larger scales [44] . This, together with the confinement of minerals to very thin nanometer dimensions, suggests that the nanocomposite in bone is a means to overcome the intrinsic limitations of each of the constituents, and to form a composite that amplifies the superior properties of the two. Our model opens a new possibility to study bone nanomechanics; for example, investigating the effect of mineral shape, size and orientation with chemical detail. In future work, the model developed here can also be applied to study brittle bone disease and other bone disorders, setting the stage for many fundamental investigations. Other future efforts could focus on further structure refinement of the model and additional experimental validation, in particular considering the distribution of mineral at larger-length scales. Model overview The goal is to develop a full-atomistic model that enables us to perform a systematic study of bone nanomechanics from a fundamental, molecular point of view. This goes beyond earlier theoretical, computational and analytical models (references and discussion see main text) that do not include the full biochemical details, and allows us to ask questions such as ‘what is the deformation mechanism in bone fibrils?’ or ‘what is the load transfer mechanism between collagen and mineral platelets?’. The geometry and composition of the model are summarized in Fig. 1b , indicating varied levels of mineral content. The 0% case corresponds to a non-mineralized collagen microfibril and also clearly shows the gap and overlap region ( Fig. 1b ) that emerges from the geometrical arrangement of collagen protein molecules. The D -period corresponds to the periodicity typically observed in collagen fibrils. The 20 and 40% mineral-density cases correspond to the two different mineral concentrations in the collagen microfibril. A recent study [30] conducted of a pure collagen fibril has shown good agreement with experimental results. This prior work forms the basis for the model of bone, accomplished here by incorporating minerals in collagen in increasing densities (as it occurs naturally during bone formation), whereas accounting for the complexity of the chemical interactions [26] , [45] , [46] , [47] that have not yet been incorporated in earlier models. Collagen protein force field parameterization Collagen is the sole protein that features hydroxyproline (HYP), a non-standard amino acid, resulting from the post-translational hydroxylation of proline. As it is rarely found, HYP is not parameterized in common biomolecular force fields, such as CHARMM [48] . However, a set for HYP has been developed [49] based on quantum mechanical models and have been subsequently used to derive the atomistic parameters that best match the quantum-mechanics calculation, with particular focus on the correct modelling of the pucker of the HYP ring. These parameters have been then successfully incorporated into an extended CHARMM force field as used for collagen modelling in a series of previous works [30] , [50] , [51] . This model is also used here. Crystal geometry and HAP force field parameterization We generated the hexagonal HAP crystal unit cell by using Material Studio 4.4 (Accelrys, Inc.), which features the following lattice parameters: a =9.4214 Å, b =9.4214 Å, c =6.8814 Å, α =90°, β =90° and γ =120°. On the basis of this unit cell (with 44 atoms per unit cell), HAP crystals of varying size are generated for the purpose of this study, using the in silico mineralization method described below. Force fields for biomaterial simulations like CHARMM [48] do not include parameters for mineral crystal, such as HAP. Therefore, to model protein–HAP composites, we extend the CHARMM force field and use bond, angle and dihedral parameters following those reported earlier [52] , which are based on both quantum mechanical calculations and empirical data. For non-bonded parameters, we adopt a Born–Mayer–Huggins model. For non-bonded terms, we use data from Bhowmik et al . [53] in which the authors fitted the Born–Mayer–Huggins potential [52] with a simpler Lennard–Jones potential. Mineralized collagen microfibril model: in silico mineralization The collagen microfibril model used here is based on Protein Data Bank entry 3HR2 that was used as a basis for the non-mineralized collagen fibril model reported in [30] . For further information, we refer the reader to a previous paper with the details on the development of the collagen fibril atomistic model [30] and to the work that describes the details of the X-ray crystallography [54] . The mineralized models are built starting from the non-mineralized model by filling the model’s periodic box of HAP unit cells. Then, the HAP unit cells that have at least one atom overlapping with the atoms of collagen are removed. In this way, the HAP is left only in void space of the collagen fibril box. The overlapping condition is controlled by a chosen cutoff distance between HAP atoms and collagen atoms. By selecting the appropriate cutoff distance, it is possible to add more or less HAP unit cells and, thus, reach varied degrees of mineralization. This procedure is implemented through a tcl script used in the Visual Molecular Dynamics programme [55] . The choice of physiologically relevant amounts of HAP is chosen based on the literature [2] , [56] , which show that the content of the mineral phase is 60–70% w/w of bone tissue. In addition to the crystallites associated with the collagen fibrils (intrafibrillar mineralization), a significant amount of mineral is believed to be located in the spaces between the fibrils (extrafibrillar mineralization). It has been reported that the extrafibrillar mineral fraction can account to as much as 75% of the total mineral in bone tissues [57] , [58] , [59] . Therefore, in our models, which account only for interfibrillar mineralization, we consider degrees of mineralization of up to 40%, which allows us to study moderately to highly mineralized fibrils. The orientation and surface of HAP crystals also has a significant effect in controlling the collagen–mineral interactions. Recent studies using density functional theory shows that the mineral crystal surface (that is, either a OH- or a Ca-terminated surface) has a significant role in controlling the interaction between collagen and HAP [60] . In our model, the mineral crystals are oriented such that orientation of the OH groups of the crystal is parallel to the collagen fibril axis as shown in Fig. 1b . This orientation of crystals and the growth of the crystals along the fibril axis typically observed in experiments [56] are, hence, consistent with our mineralized collagen microfibril model. The mineral distribution inside the unit cell and its densities are shown in Fig. 2a . To enable a direct comparison with experimental results for mineral distribution, we utilize the density distribution for non-mineralized and mineralized collagen as reported in Nudelman et al . [26] , and plot the difference of the two data sets in comparison with our 40% mineral-density case ( Fig. 2c ). It is important to note that the in vivo mineralization process is a very complex phenomenon, in which immature amorphous HAP clusters nucleate close to the C-terminal end (which is at the gap-to-overlap transition region), and then grow by further mineral deposition. Furthermore, the process is believed to be assisted by acidic non-collagenous proteins. This process is too complex to be reliably replicated with direct atomistic simulations. Hence, our approach is to mimic the mineralization process by filling the void space within the collagen unit cell, in the process described above. Future works could be devoted to improve the in silico model of the mineralization process, to mimic more closely the in vivo mature mineralization state. Fibril equilibration Molecular dynamics simulations are performed using the LAMMPS code [61] and the modified CHARMM force field described above. The constructed collagen–HAP model is first geometrically optimized through energy minimization, and then an NVT equilibration is performed for 2 ns. The unit cell that comprises collagen and HAP has triclinic symmetry as described in earlier work [54] . Rigid bonds are used to constrain covalent bond lengths, thus allowing for an integration time step of 2 fs. Non-bonding interactions are computed using a switching function between 0.8 and 1.0 nm for van der Waals interactions, whereas the Ewald summation method [62] is applied to describe electrostatic interactions. The system temperature is maintained at 300 K (room temperature). We confirmed that the root mean square deviation of the mineralized collagen is stable, and that no major changes occur in the structure towards the end of equilibration. In silico mechanical testing To assess the mechanical properties of mineralized collagen fibrils, we perform stress-controlled ( NP ij T ) molecular dynamics simulations with increasing tensile stress applied along the x axis of the unit cell as depicted in Fig. 3a . The unit cell is under constant atmospheric pressure along other two axes (y and z). We use an NP ij T ensemble [63] for loading the samples with different stress states ( σ =− P ij ) ranging from: (i) atmospheric pressure, (ii) 20 MPa, (iii) 60 MPa and (iv) 100 MPa. We observe that samples reached equilibration under applied load at ~6 ns. The strain is computed as ε= ( L−L o )/ L o , where L o is the equilibrium length identified at atmospheric pressure. To ensure that equilibrium is achieved, we monitor the pressure at equilibrium, root mean square deviation, and confirm that the size of the simulation cell reaches a steady-state value. Using the fibril strain ε associated with each applied stress σ , we obtain the stress–strain behaviour for each case by plotting σ over ε . We use a second-order polynomial function to fit the stress–strain data, which includes all positive coefficients. The general form of the equation is σ=a 1 ε 2 + a 2 ε . For both non-mineralized and mineralized data sets, the coefficients a 1 and a 2 are positive so that the fitting procedure is consistent. The modulus is computed from the first derivative of a polynomial function that is fitted to the stress–strain data. The polynomial functions that are used to fit the stress–strain data are as follows: (a) for the 0% case, 2874.9 x 2 +240.61 x ; (b) for the 20% case, 8101.8 x 2 +787.89 x ; and (c) for the 40% case, 13651 x 2 +1094.2 x (with appropriate dimensions to express stress in MPa).The computational time requirement for equilibration is 0.2 ns per week using 24 processors for the 40% mineral-density case. Visualization We use Visual Molecular Dynamics [55] to visualize the snapshots of simulation and compute hydrogen bonds. We count the hydrogen bonds within a cutoff distance of 3.5 Å and an angle range of 30°. MATLAB (MathWorks, Inc.) is used to plot the stress distribution inside the collagen microfibril model. Strain analysis We find the distance between the centre of mass of glycine residues in each chain of the collagen triple helix, and then utilize the distance between the centre of mass to compute the total deformation in collagen microfibril. This approach of computing the strain in a collagen molecule has been discussed in detail in earlier work [64] , and the readers are referred to this article for further information. Once the deformation is obtained for the whole microfibril, we compute the deformation of the gap and overlap region. Theoretical models We compare the effective modulus predicted by atomistic simulations with analytical models by Halpin–Tsai [36] , [38] and Gao et al . [37] , and also with the experimental values reported in Hang and Barber [31] . According to the Halpin–Tsai model, the longitudinal modulus of a unidirectional plane, parallel platelet-reinforced composite is given by where E m is the matrix modulus (here we use 0.5 GPa as the value obtained from our non-mineralized sample) and Φ is the mineral volume fraction. The constants A and B are given by where ρ is the aspect ratio of the mineral (for biological materials, such as bone ρ~ 30) and E p is the modulus of the mineral platelet (100 GPa). According to Gao et al . [37] , the effective modulus for a nanocomposite is given by where Φ is the mineral volume fraction, E mg is the elastic modulus of mineral (100 GPa), ρ is the aspect ratio of the mineral (for bone ρ~ 30) and G p =0.03 GPa is the shear modulus of collagen. The comparison of the analytical models, simulation and experiments are shown in Fig. 7 . Force field files, scripts and atomic structure files The force-field files for LAMMPS, structure files in PDB format and all scripts used in this study are available from the corresponding author upon request. How to cite this article : Nair, A. K. et al . Molecular mechanics of mineralized collagen fibrils in bone. Nat. Commun. 4:1724 doi: 10.1038/ncomms2720 (2013).